ε-Iron carbide as a low-temperature Fischer–Tropsch synthesis catalyst ε -Iron carbide has been predicted to be promising for low-temperature Fischer–Tropsch synthesis (LTFTS) targeting liquid fuel production. However, directional carbidation of metallic iron to ε -iron carbide is challenging due to kinetic hindrance. Here we show how rapidly quenched skeletal iron featuring nanocrystalline dimensions, low coordination number and an expanded lattice may solve this problem. We find that the carbidation of rapidly quenched skeletal iron occurs readily in situ during LTFTS at 423–473 K, giving an ε -iron carbide-dominant catalyst that exhibits superior activity to literature iron and cobalt catalysts, and comparable to more expensive noble ruthenium catalyst, coupled with high selectivity to liquid fuels and robustness without the aid of electronic or structural promoters. This finding may permit the development of an advanced energy-efficient and clean fuel-oriented FTS process on the basis of a cost-effective iron catalyst. In the foreseeable future, transportation fuel will remain carbon based. Fischer–Tropsch synthesis (FTS) is a key technology in heterogeneous catalysis for the production of chemicals including liquid fuel from carbon sources alternative to unsustainable crude oil [1] , [2] , [3] , [4] . The wide availability and resistance to poisons, high adaptability to broad H 2 /CO ratios and versatility to various useful products make iron-based catalysts ideal for converting H 2 -deficient syngas (CO and H 2 ) from coal and renewable biomass. During FTS, carbon atoms cleaved from CO show high affinity to iron atoms, so iron catalysts present rich phase chemistry towards the formation of iron carbide(s) [5] . While cementite ( θ -Fe 3 C) and Hägg carbide ( χ -Fe 5 C 2 ) are mostly reported in FTS studies, hexagonal iron carbides ( ε ′-Fe 2.2 C, ε -Fe 2 C) are sporadically identified at comparatively low temperatures and/or low H 2 /CO ratios [6] , [7] , [8] , [9] , [10] , [11] . These iron carbides differ from carbon positions in the hexagonally close packed iron lattice. The carbon atoms in θ -Fe 3 C and χ -Fe 5 C 2 are situated in trigonal prismatic (TP) interstices. The trigonal prisms are similar, but the ways for their organization in θ -Fe 3 C and χ -Fe 5 C 2 (TP-carbides) are different [12] . For ε ′-Fe 2.2 C and ε -Fe 2 C, the carbon atoms are situated in octahedral (O) interstices [5] , so they are also termed as O-carbides. The extent of structural deformation for these iron carbides increases with carbon content from θ -Fe 3 C (25 at.%) to ε -Fe 2 C (33.3 at.%). 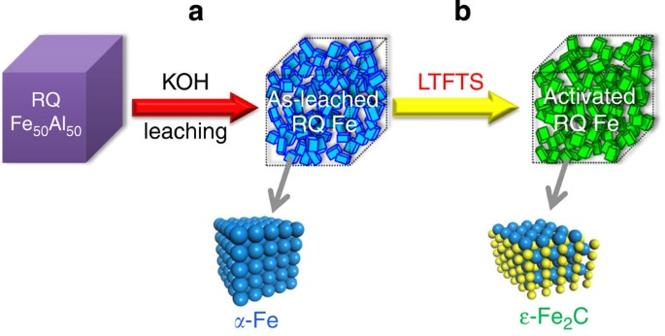Figure 1: Scheme for the preparation ofε-Fe2C from the RQ Fe50Al50alloy. (a) Alkali leaching of the RQ Fe50Al50alloy to the skeletal RQ Fe that is constituted by theα-Fe nanocrystals. (b) On site carbidation of RQ Fe in LTFTS to the activated RQ Fe catalyst that is constituted by theε-Fe2C nanocrystals. Detailed crystal structure parameters of these iron carbides are compiled in Supplementary Table 1 . It is generally acknowledged that iron carbides, as well as in some reports, metallic iron, are the active phase in FTS [5] , [10] , [13] , [14] , [15] , [16] , [17] , [18] , [19] , [20] . At typical FTS temperature of 543 K, many reports agree that the active phase is χ -Fe 5 C 2 , while θ -Fe 3 C is a spectator or a deactivation phase [10] , [19] , [21] , [22] , [23] . Pure χ -Fe 5 C 2 nanoparticles (NPs) have been synthesized and supported, and proven to be better than a reduced haematite catalyst in terms of CO conversion and product selectivity [24] . In contrast, O-carbides are favoured in high carbon potential ( μ c ) surroundings, that is, low temperature (<473 K) and high CO partial pressure, with μ c more sensitive to temperature than to pressure [25] . However, kinetic factors (lattice deformation, carbon diffusion) are adverse to their formation at low temperature. Unfortunately, at elevated temperatures, O-carbides readily evolve into TP carbides [9] , [13] . Attractively, a recent theoretical study illustrated that the barriers on Fe 2 C for CO dissociation and hydrogenation are both the lowest amongst Fe 2 C(011), Fe 5 C 2 (010), Fe 3 C(001) and Fe 4 C(100) (not found in FTS [25] ) surfaces with carbon vacancies [26] . According to a volcano-plot for metal–CO bond strength versus FTS activity for iron and cobalt [27] , increasing the carbon content in iron carbide will weaken the Fe–CO bonding and hence enhance the activity. These works prompt us to develop a new catalytic material that is constituted by ε -Fe 2 C holding promise as an active catalyst in LTFTS. However, how to lift the kinetic hindrances on ε -Fe 2 C formation imposed by the low temperature for ensuring a high μ c while the low temperature is indispensible to stabilize this phase seems an insurmountable dilemma. We demonstrate here that by exploiting the highly reactive rapidly quenched skeletal iron (RQ Fe) as the catalyst precursor, this dilemma can be neatly disentangled. We succeed in synthesizing an iron catalyst that is constituted by ε -Fe 2 C nanocrystals, and disclose for the first time its exceptional catalytic behaviour in LTFTS. Structural characteristics of RQ Fe The RQ Fe is prepared by alkali leaching of aluminum from a binary rapidly quenched Fe 50 Al 50 alloy (Fe/Al, w / w ) solidified at a cooling rate of ~3 × 10 7 K s −1 . The preparation procedures of the RQ Fe 50 Al 50 alloy and RQ Fe have been described elsewhere [28] . Because of the extremely high solidification speed, the long-range diffusion of the atoms in the melt is retarded, so the atoms are frozen before they relax freely to the equilibrium position [29] . As a result, the grains in the rapidly quenched alloys are nanocrystalline and abundant in low-coordination sites [30] , [31] . Dissolving the sacrificial metal, for example, aluminum in RQ Fe 50 Al 50 , can further reduce the grain size as well as the coordination number. These peculiar structural characteristics are expected to lower the barrier for the activation of metallic iron to ε -Fe 2 C ( Fig. 1 ). Figure 1: Scheme for the preparation of ε -Fe 2 C from the RQ Fe 50 Al 50 alloy. ( a ) Alkali leaching of the RQ Fe 50 Al 50 alloy to the skeletal RQ Fe that is constituted by the α -Fe nanocrystals. ( b ) On site carbidation of RQ Fe in LTFTS to the activated RQ Fe catalyst that is constituted by the ε -Fe 2 C nanocrystals. 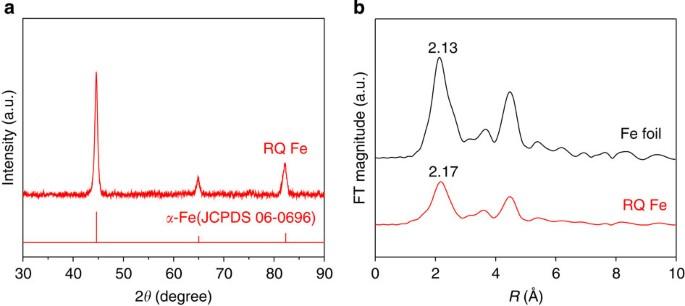Figure 2: Microstructure of the as-leached RQ Fe. (a) Powder XRD pattern of the as-leached RQ Fe that is indexable to body centred cubic (bcc)α-Fe (JCPDS 06-0696); the crystallite size of metallic iron in the as-leached RQ Fe is estimated to be 13.5 nm based on the Scherrer equation and the broadening of the primary (110) diffraction peak at 2θof 44.6°. (b) Fourier-transformed Fe K-edge EXAFS patterns of the as-leached RQ Fe and the reference Fe foil. Full size image Figure 2a shows that there are only features at 2 θ of 44.6, 64.8 and 82.2° in the X-ray diffraction (XRD) pattern of the as-leached RQ Fe, assignable to body centred cubic α -Fe (JCPDS 06-0696). The metallic iron nanocrystals constituting the RQ Fe are as small as 13.5 nm. It is noteworthy that the 2 θ values of RQ Fe is slightly but reproducibly smaller than the standard values, indicating the occurrence of lattice expansion owing to confined relaxation of the iron atoms, as also observed on RQ Ni prepared by the same technique [32] . This finding is consistent with Fourier transforms of the k 1 -weighted Fe K-edge extended X-ray absorption fine structure (EXAFS) data in Fig. 2b and Table 1 . EXAFS indicates that RQ Fe has a longer Fe–Fe coordination distance (2.50 Å) than the Fe foil (2.48 Å), with the latter being identical to that of the α -Fe standard [33] . Moreover, the radial distribution function (RDF) of RQ Fe displays markedly lower peak amplitudes than the Fe foil, which signifies its lower coordination number. It is true that the Fe–Fe coordination number of RQ Fe is only 4.0, while that of the Fe foil is 8.0, inferring that the as-leached RQ Fe is highly reactive. Figure 2: Microstructure of the as-leached RQ Fe. ( a ) Powder XRD pattern of the as-leached RQ Fe that is indexable to body centred cubic ( bcc ) α -Fe (JCPDS 06-0696); the crystallite size of metallic iron in the as-leached RQ Fe is estimated to be 13.5 nm based on the Scherrer equation and the broadening of the primary (110) diffraction peak at 2 θ of 44.6°. ( b ) Fourier-transformed Fe K-edge EXAFS patterns of the as-leached RQ Fe and the reference Fe foil. Full size image Table 1 The Fe K-edge EXAFS fit data of the RQ Fe and the Fe foil. Full size table Structure determination of ε -Fe 2 C After being subjected to LTFTS at 443 K for 20 min in a batchwise reactor (30 bar at RT, H 2 /CO/N 2 =64/32/4 by volume, polyethylene glycol (PEG200, M w =200) as the reaction medium [34] , [35] ), the phase composition was examined on a synchrotron radiation diffractometer, which is well suited to study the weak diffractions of iron carbides than on conventional diffractometer [12] . In the synchrotron XRD pattern shown as Fig. 3a , aside from a small feature at 2 θ of 44.6° due to remainder metallic iron, new peaks emerge at 2 θ of 37.3, 41.4, 43.0 and 56.9°, which are indexable to the (100), (002), (101) and (102) reflections of either ε ′-Fe 2.2 C or ε -Fe 2 C (JCPDS 36-1249), respectively. The two O-carbides have similar crystallographic structure and are difficult to differentiate solely by XRD [7] , [10] , [11] , [25] , so we temporarily refer to this phase as O-carbide. The crystallite size of the O-carbide (8.1 nm) is smaller than that of the as-leached RQ Fe. No magnetite (Fe 3 O 4 ) is identified. It is impressive that RQ Fe has been carbidized predominantly to O-carbide on site at 443 K within 20 min, which would otherwise be hindered by the low temperature [25] . We believe that the highly coordinatively unsaturated microstructure of the as-leached RQ Fe is essential for the facile low-temperature carbidation. Its small crystallite size and expanded lattice favour the fast diffusion of carbon atoms into the bulk and hence the thorough carbidation. Lattice expansion may additionally facilitate the accommodation of the carbon atoms and lower the deformation energy. Note that among the iron carbides, the O-carbides have the highest degree of deformation of the iron lattice associated with the highest carbon content [25] . Supplementary Figure 1 also shows that the O-carbide is the predominant phase in the RQ Fe after LTFTS at 473 and 423 K. Furthermore, in situ XRD characterization under conditions close to those for LTFTS at 443 K is carried out, which testifies the phase transformation from α -Fe to O-carbide. The latter, once formed, is highly stable with the reaction time at 443 K in syngas ( Supplementary Figs 2 and 3 ). 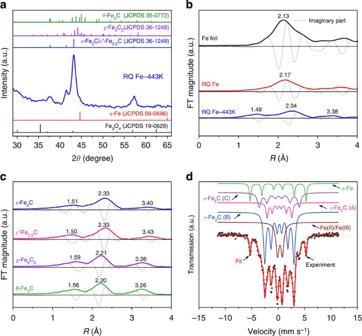Figure 3: The structure of the RQ Fe after LTFTS at 443 K. (a) Synchrotron radiation XRD pattern of the RQ Fe after LTFTS; all peaks can be indexed to the O-carbide phase (ε′-Fe2.2C orε-Fe2C, JCPDS 36-1249); the crystallite size of the O-carbide is estimated to be 8.1 nm based on the Scherrer equation and the broadening of the primary (101) diffraction peak at 2θof 43.0°. (b) Experimental Fourier-transformed Fe K-edge EXAFS pattern of the RQ Fe after LTFTS, along with those of the as-leached RQ Fe and the reference Fe foil for comparison. The imaginary parts of the Fourier-transformed data are plotted as dashed lines. (c) Theoretical Fourier-transformed EXAFS patterns forε-Fe2C,ε′-Fe2.2C,χ-Fe5C2andθ-Fe3C simulated using the FEFF8.2 code based on the structural parameters compiled inSupplementary Table 1. The imaginary parts of the Fourier-transformed data are plotted as dashed lines. (d)57Fe Mössbauer spectrum of the RQ Fe after LTFTS; the on site activated catalyst contains 73.1% ofε-Fe2C, 9.4% ofα-Fe and 17.5% of the Fe(II)/Fe(III) species, verifying that the metallic iron in RQ Fe can be effectively carbidized toε-Fe2C during LTFTS. Figure 3: The structure of the RQ Fe after LTFTS at 443 K. ( a ) Synchrotron radiation XRD pattern of the RQ Fe after LTFTS; all peaks can be indexed to the O-carbide phase ( ε ′-Fe 2.2 C or ε -Fe 2 C, JCPDS 36-1249); the crystallite size of the O-carbide is estimated to be 8.1 nm based on the Scherrer equation and the broadening of the primary (101) diffraction peak at 2 θ of 43.0°. ( b ) Experimental Fourier-transformed Fe K-edge EXAFS pattern of the RQ Fe after LTFTS, along with those of the as-leached RQ Fe and the reference Fe foil for comparison. The imaginary parts of the Fourier-transformed data are plotted as dashed lines. ( c ) Theoretical Fourier-transformed EXAFS patterns for ε -Fe 2 C, ε ′-Fe 2.2 C, χ -Fe 5 C 2 and θ -Fe 3 C simulated using the FEFF8.2 code based on the structural parameters compiled in Supplementary Table 1 . The imaginary parts of the Fourier-transformed data are plotted as dashed lines. ( d ) 57 Fe Mössbauer spectrum of the RQ Fe after LTFTS; the on site activated catalyst contains 73.1% of ε -Fe 2 C, 9.4% of α -Fe and 17.5% of the Fe(II)/Fe(III) species, verifying that the metallic iron in RQ Fe can be effectively carbidized to ε -Fe 2 C during LTFTS. Full size image To discern the identity of the O-carbide, the RQ Fe after LTFTS at 443 K was further characterized by Fe K-edge EXAFS. Figure 3b shows that the RDF of the RQ Fe after LTFTS is at sharp variance with that of the as-leached RQ Fe or the Fe foil, which is consistent with the XRD observation that only little metallic iron is survived. The fitted structural parameters are summarized in Supplementary Table 2 . As there are no authentic TP- and O-carbide standards, their RDFs are simulated for a direct visual comparison ( Fig. 3c ). TP-carbides and O-carbides can be easily distinguished by the longer first Fe–C shell distances and the shorter first and second Fe–Fe shell distances of the former. The experimental RDF of the RQ Fe after LTFTS resembles the simulated ones of the O-carbides, so the possibility of TP-carbides is ruled out. Although the first Fe–C and Fe–Fe shell distances of the two O-carbides are quite similar, Fig. 3c hints that one can distinguish them by the shorter second Fe–Fe shell distance for ε -Fe 2 C (3.40 Å). Figure 3b shows that the second Fe–Fe shell distance of the RQ Fe after FTS is located at 3.38 Å, which prefers the assignment to ε -Fe 2 C. 57 Fe Mössbauer spectroscopy is a powerful tool to identify and quantify the iron phases formed during FTS. Figure 3d presents the 57 Fe Mössbauer spectrum of the RQ Fe after LTFTS at 443 K and the deconvoluted sub-spectra; the corresponding parameters are listed in Table 2 . Metallic iron is identified based on the small sextet with the hyperfine magnetic field ( H ) of 329 kOe (ref. 8 ). The formation of ε -Fe 2 C is corroborated by three sextets with H values of 142 (Sextet A), 172 (Sextet B) and 235 kOe (Sextet C) [6] , [36] , [37] . The intensity ratio of A: B: C is close to the theoretical ratio of 1: 4: 1.6 corresponding to the population of the individual crystallographic sites in the ε -Fe 2 C lattice [6] . In contrast, if the O-carbide was ε ′-Fe 2.2 C, there should only be one sextet [6] , [7] , [13] , [34] . No sextets with H values of ~460 and 490 kOe are found, verifying the absence of Fe 3 O 4 (ref. 38 ). Rather, there is a superparamagnetic (spm) doublet with the isomer shift (IS) of 0.34 mm s −1 and the quadrupole splitting (QS) of 0.92 mm s −1 attributable to Fe(II) or Fe(III) species [39] , [40] , which may be due to the presence of some poorly crystallized iron oxide. Assuming the same recoil-free factors, the contents of the iron species in the RQ Fe after FTS are proportional to their respective integral areas. Hence, one can figure out that there is only 9.4% of metallic iron, 17.5% of the Fe(II)/Fe(III) species and as high as 73.1% of ε -Fe 2 C. Table 2 57 Fe Mössbauer parameters of the RQ Fe after LTFTS. Full size table LTFTS activity As pointed out by Kou and coworkers, the high temperature (503 K and above) currently used is not demanded by the very exothermic FTS reaction itself, but by activation of the iron catalysts [35] . We find that our ε -Fe 2 C-dominant RQ Fe catalyst is highly active in LTFTS at 443 K, 60 K lower than the industrial iron-based LTFTS process [41] , which was first developed by Lurgi and Ruhrchemie in 1955 on fixed-bed multitubular ARGE reactors followed by Sasol in 1993 according to their own design of the bubble column reactor over a precipitated iron-based catalyst [42] . The catalytic results listed in Table 3 show that the initial catalytic activity ( r 0 ) is 43 mol CO mol Fe −1 h −1 ( Table 3 , entry 2). This value is approximately one-to-two magnitudes higher than the activities of a noble 5%Ru/SiO 2 catalyst at 473 K ( Supplementary Table 3 , entry 1) [43] . As the highest LTFTS activity ever reported on a ruthenium nanocluster catalyst was calculated at the CO conversion of ~75% (ref. 44 ), we analogously calculated the activity of the RQ Fe catalyst at a similar CO conversion. It is remarkable that the activity of the RQ Fe catalyst at 443 K ( Supplementary Table 3 , entry 3) is comparable to that of the ruthenium nanocluster catalyst at 423 K ( Supplementary Table 3 , entry 2). Although the reaction temperature for the former is 20 K higher, iron is advantageous in that it is four orders of magnitude cheaper than ruthenium [45] . When the reaction temperature is elevated to 473 K, the r 0 of the RQ Fe catalyst is further increased to 71 mol CO mol Fe −1 h −1 ( Table 3 , entry 3). Moreover, the RQ Fe catalyst remains highly active even when further lowering the temperature to 423 K, giving rise to an r 0 of 16 mol CO mol Fe −1 h −1 ( Table 3 , entry 1), which conforms to the observation that carbidation can occur at as low as 423 K (ref. 46 ). Table 3 Catalytic activities in LTFTS*. Full size table The activity of the RQ Fe catalyst is substantially higher than the best results ever reported on iron catalysts in LTFTS. It was reported that on an amorphous Fe-W nanocatalyst prepared by reducing FeCl 3 with KBH 4 in water, the CO activity was 0.83 mol CO mol Fe −1 h −1 at 473 K ( Supplementary Table 3 , entry 4) [34] , which is one-seventh of the value over the RQ Fe catalyst at the same temperature and similar conversion ( Supplementary Table 3 , entry 5). On an amorphous Fe nanoparticle (NP) catalyst prepared by reducing FeCl 2 with NaBH 4 in ethylene glycol–water, an improved activity of 1.5 mol CO mol Fe −1 h −1 was reported at 423 K ( Supplementary Table 3 , entry 6) [35] , but it is still substantially lower than that over the RQ Fe catalyst at the corresponding temperature and similar conversion ( Supplementary Table 3 , entry 7). The lower activity of the two borohydride-reduced iron catalysts is possibly due to the existence of alloying boron that severely hinders the carbidation of iron at low temperature, and, indeed, for the amorphous Fe NPs catalyst after LTFTS, the diffractions of the iron carbide were much weaker than those of metallic iron [35] . This may be analogous to the impeding effect of the alloying nickel on the bulk carbidation of iron observed by Raupp and Delgass [6] . The ε -Fe 2 C-dominant RQ Fe catalyst also outperforms the crystalline Fe NPs catalyst prepared according to ref. 47 by reducing FeCl 3 with N 2 H 4 ·H 2 O and the Fe–Cu–K–Si catalyst prepared according to ref. 10 by coprecipitation in LTFTS. We find that the crystalline Fe NPs catalyst and the Fe–Cu–K–Si catalyst show low activities at 443 K ( Table 3 , entries 4 and 5). The poor activity of the former may be caused by its large crystallite size (33.2 nm, Supplementary Fig. 6a ) that is adverse to carbidation, as evidenced by the barely visible feature of O-carbide after LTFTS ( Supplementary Fig. 7a ). The crystallite size of metallic iron on the Fe–Cu–K–Si catalyst is 8.6 nm ( Supplementary Fig. 6b ), which is even smaller than that of the as-leached RQ Fe. However, most of metallic iron in this catalyst remains intact after LTFTS, aside from less intense features of Fe 3 O 4 and O-carbide ( Supplementary Fig. 7b ). We propose that the strong promoter–iron interaction in this multiply promoted catalyst stabilizes the metallic iron NPs by lowering the surface energy [48] , which alters the tendency of carbidation despite of its small size. As χ -Fe 5 C 2 is well known as the active phase in FTS above 473 K (refs 10 , 23 , 24 ), according to ref. 25 we synthesized the χ -Fe 5 C 2 -dominant RQ Fe catalyst (denoted as RQ Fe- χ ) with the crystallite size and surface area similar to the ε -Fe 2 C-dominant RQ Fe catalyst ( Supplementary Fig. 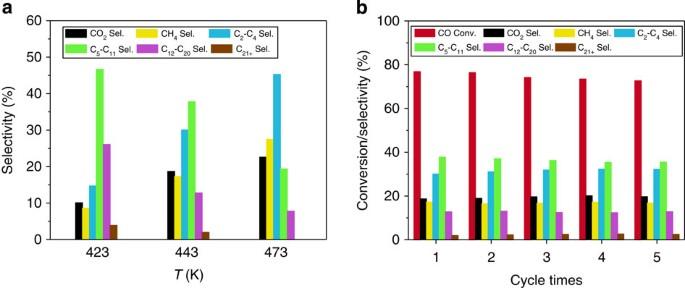Figure 4: Catalytic results over the RQ Fe catalyst in LTFTS. (a) The CO2selectivities and the distributions of hydrocarbons over the RQ Fe catalyst in LTFTS conducted at 423, 443 and 473 K; other reaction conditions:P=30 bar at RT, H2/CO/N2=64/32/4, 4.48 mmol Fe, 20 ml PEG200, and stirring rate of 800 r.p.m.; the products shift to longer hydrocarbons with the decrease in the reaction temperature from 473 to 423 K. (b) CO conversion and product distribution over the RQ Fe catalyst in five successive LTFTS cycles; reaction conditions:T=443 K,P=30 bar at RT, H2/CO/N2=64/32/4, 4.48 mmol Fe, 20 ml PEG200 and stirring rate of 800 r.p.m.; after each catalytic run, the catalyst is simply separated from the liquid phase by a magnet, followed by washing with ethanol and PEG200 twice. The recovered catalyst is reused without reactivation. The hydrocarbon selectivities are normalized with the exception of CO2. 8 and Supplementary Table 4 ). Under identical reaction conditions at 443 K, the r 0 of the RQ Fe- χ catalyst ( Table 3 , entry 6) is only about 25% of that of the ε -Fe 2 C-dominant RQ Fe catalyst, which is consistent with theoretical predictions that ε -Fe 2 C is more active than χ -Fe 5 C 2 in FTS [25] , [27] . Besides the iron-based catalysts, the RQ Co and amorphous Co–B [49] catalysts are prepared and evaluated in LTFTS at 443 K. The r 0 of the RQ Co catalyst ( Table 3 , entry 7) is higher than that of the Co–B catalyst ( Table 3 , entry 8), but is still appreciably lower than that over the RQ Fe catalyst at the same temperature. These results are in agreement with previous observations [35] , [50] and can be explained as a result of the lower activation energy on iron than on cobalt for FTS [51] . Selectivity and stability When lowering the FTS temperature, the chain growth probability, α, will increase, favouring the production of high-value long-chain hydrocarbons [41] . Figure 4a presents the temperature-dependent product distributions over the RQ Fe catalyst. The selectivities of the hydrocarbons at different temperatures follow the Anderson−Schulz−Flory (ASF) distribution ( Supplementary Fig. 9 ), with the α-value increasing as anticipated from 0.71 to 0.79 with the decrease in the temperature from 473 to 423 K. Meanwhile, the selectivity to CO 2 evolves in an opposite trend from 22.6 to 10.1%. According to Fig. 4a , at 473 K, the low-value CH 4 and C 2 –C 4 hydrocarbons are the primary products. At 443 K, the C 2 –C 4 and C 5 –C 11 (gasoline fraction) hydrocarbons become dominant. At 423 K, the sum of the gasoline fraction and C 12 –C 20 hydrocarbons (diesel fraction) amounts to 73%, with a small amount of the C 21+ products. It was reported that on the amorphous Fe NPs catalyst and at 423 K, the selectivity to C 5+ hydrocarbons is 56% with the α-value of 0.72 (ref. 35 ), showing that ε -Fe 2 C is intrinsically excellent in producing transportation fuels. Figure 4: Catalytic results over the RQ Fe catalyst in LTFTS. ( a ) The CO 2 selectivities and the distributions of hydrocarbons over the RQ Fe catalyst in LTFTS conducted at 423, 443 and 473 K; other reaction conditions: P =30 bar at RT, H 2 /CO/N 2 =64/32/4, 4.48 mmol Fe, 20 ml PEG200, and stirring rate of 800 r.p.m. ; the products shift to longer hydrocarbons with the decrease in the reaction temperature from 473 to 423 K. ( b ) CO conversion and product distribution over the RQ Fe catalyst in five successive LTFTS cycles; reaction conditions: T =443 K, P =30 bar at RT, H 2 /CO/N 2 =64/32/4, 4.48 mmol Fe, 20 ml PEG200 and stirring rate of 800 r.p.m. ; after each catalytic run, the catalyst is simply separated from the liquid phase by a magnet, followed by washing with ethanol and PEG200 twice. The recovered catalyst is reused without reactivation. The hydrocarbon selectivities are normalized with the exception of CO 2 . Full size image The high activity of the RQ Fe catalyst allows the use of compact reactors and mild operation conditions, and the high selectivity to transportation fuels simplifies subsequent product purification, which are very attractive for the development of an iron-based advanced FTS process. However, the iron-based catalysts, when in the absence of promoter(s), are usually notorious for their high deactivation rates, which has been a main concern of industrial research [5] . Therefore, the recyclability and stability of the RQ Fe catalyst in LTFTS at 443 K is examined. Figure 4b shows that the CO conversion decreases only by 4.2% from the first run to the fifth run. The ~1% per run activity drop may be due to small catalyst loss during recovery, for the recovery procedures have not been elaborately optimized. This possibility is supported by the virtually unchanged product distributions also depicted in Fig. 4b , which shows that the nature of the catalyst does not change during the recycling and stability test. The synchrotron XRD pattern of the RQ Fe catalyst after the stability test ( Supplementary Fig. 10 ) confirms that ε -Fe 2 C remains as the dominant phase. The same conclusion is held when the cycle time is further increased to 27 runs ( Supplementary Figs 11 and 12 ). Aside from the theoretical prediction that ε -Fe 2 C is the thermodynamically most stable iron carbide among the TP- and O-carbides at low temperature [25] , it has been reported that iron catalysts with smaller particles are desirably more resistant to oxidation by CO 2 and water produced during FTS [6] , which may be the physical origin of the high robustness of the RQ Fe catalyst constituted by nanocrystalline ε -Fe 2 C. We are uncertain at present whether ε -Fe 2 C is inherently more resistant to oxidation, although ref. 52 found that ε ′-Fe 2.2 C, another O-carbide, appears to be less susceptible to oxidizing conditions than χ -Fe 5 C 2 . Nevertheless, the possible inhibition of water on the LTFTS activity of ε -Fe 2 C due to water accumulation at longer reaction times requires further exploration in a continuous-flow reactor. Sintering usually does not play a significant role in the deactivation of the iron catalysts under typical FTS temperatures [5] , so it is unlikely to operate at much lower temperature employed in the present case. In conclusion, we demonstrate that the ε -Fe 2 C-dominant catalyst can be successfully prepared by on site carbidation of RQ Fe during LTFTS. The structural peculiarities of the RQ Fe (low coordination number, nanoscale and expanded lattice) are essential to overcome the seemingly insurmountable hindrance that the carbidation of metallic iron to ε -Fe 2 C is kinetically limited at low temperature, whereas the ε -Fe 2 C phase is stable only at low temperature. We identify that the ε -Fe 2 C phase exhibits excellent activity at as low as 423 K, high selectivity to transportation fuels and remarkable robustness in stability tests, making it a highly attractive candidate for practical applications. This work heralds the coming of an energy-efficient and clean transportation fuel-oriented LTFTS process with the high-performance while cost-effective ε -Fe 2 C catalyst as the kernel, which promises to be one of the most important advances in the LTFTS study. Preparation of RQ Fe Previous studies revealed that in FTS at 543 K, the Raney Fe derived from the Raney Fe 50 Al 50 alloy is more active than those prepared from other alloy compositions [53] , whereas the former is inferior to the RQ Fe derived from the RQ Fe 50 Al 50 alloy [28] . Therefore, the RQ Fe 50 Al 50 alloy is an ideal starting material to prepare the active iron catalyst for LTFTS. The RQ Fe 50 Al 50 alloy (Fe/Al, w / w ) was prepared by the single roller melt-spinning method [28] . The alloy ribbons with a cross-section of ~0.02 × 2 mm 2 were ground, sieved and the 40–80-mesh fraction was used. All other chemicals were used without further purification. The details in the chemicals were available in Supplementary Methods . According to our previous work [28] , 1 g of the RQ Fe 50 Al 50 alloy was added to a solution of KOH (2.5 g in 6.0 ml water) at 343 K under gentle stirring. After addition, the mixture was stirred at that temperature for 1 h for further alkali leaching. The black powders were collected from the solution by a magnet and washed thrice with distilled water, twice with ethanol, twice with PEG200 and finally stored in PEG200 for characterization and catalytic testing. The composition in molar ratio of the RQ Fe is 92.7Fe/7.3Al as determined by the inductively coupled plasma-atomic emission spectroscopy (ICP–AES; Thermo Elemental IRIS Intrepid). Preparation of crystalline Fe NPs The crystalline Fe NPs catalyst was prepared following the procedures proposed by ref. 47 . An amount of 4.24 g of KOH and 6.1 ml of N 2 H 4 ·H 2 O (80 wt%) was added into the FeCl 3 solution (2.42 g FeCl 3 ·6H 2 O in 12.1 ml ethanol). The mixture was stirred vigorously to homogeneity at RT and then transferred into a 50 ml stainless steel autoclave that was equipped with a manometer. The autoclave was sealed, maintained at 353 K and 60 bar (autogenous pressure) for 10 h, and then cooled naturally down to RT. The black Fe NPs were collected from the solution by a magnet and washed thrice with distilled water, twice with ethanol, twice with PEG200 and finally stored in PEG200 for characterization and catalytic testing. Preparation of Fe–Cu–K–Si The Fe–Cu–K–Si catalyst was prepared by the coprecipitation method [10] . An amount of 25.0 g of Fe(NO 3 ) 3 ·9H 2 O and 1.2 g of Cu(NO 3 ) 2 ·3H 2 O were dissolved in 100 ml of distilled water. After the solution was heated to its boiling point, near boiling Na 2 CO 3 aqueous solution (25.0 g in 100 ml water) was added dropwisely under vigorous stirring. The resulting precipitate was filtered and washed with distilled water until the pH of ~7. The washed precipitate was re-slurried in 200 ml of distilled water, and 1.9 g of K 2 SiO 3 · x H 2 O was added to the slurry under vigorous stirring. Then, 1.5 ml of concentrated HNO 3 was added to precipitate SiO 2 . The precipitate was filtered and dried at 378 K for 16 h, and then calcined in air at 573 K for 5 h at a heating rate of 5 K min −1 . The relative molar composition of the Fe–Cu–K–Si catalyst is 76.5 Fe/6.3 Cu/3.7 K/13.5 Si as determined by ICP–AES. Before characterization and catalytic testing, 0.43 g of the Fe–Cu–K–Si catalyst (4.48 mmol Fe, 100–200 mesh) was reduced at 673 K for 8 h in a 5% H 2 /Ar atmosphere with a flow rate of 40 ml min −1 at a heating rate of 10 K min −1 . After reduction, the catalyst was stored in PEG200. Preparation of RQ Fe-χ The χ -Fe 5 C 2 -dominant RQ Fe catalyst (denoted as RQ Fe- χ ) was prepared by CO treatment according to ref. 25 . An amount of 0.25 g of the RQ Fe catalyst (4.48 mmol Fe) was heated at 523 K for 2 h in 99.999% CO atmosphere with a flow rate of 20 ml min −1 at a heating rate of 2 K min −1 . After this treatment, the obtained RQ Fe- χ catalyst was stored in PEG200. Preparation of RQ Co An amount of 1.32 g of the RQ Co 40 Al 60 alloy was added to a KOH aqueous solution (3.96 g in 9.5 ml water) at 343 K under gentle stirring. After addition, the mixture was stirred at 343 K for additional 1 h for further alkali leaching. The black powders were collected from the solution by a magnet and washed thrice with distilled water, twice with ethanol, twice with PEG200 and finally stored in PEG200 for catalytic testing. The relative molar composition of the RQ Co catalyst was 93.1 Co/6.9 Al as determined by ICP–AES. Preparation of amorphous Co–B The amorphous Co–B catalyst was prepared by the chemical reduction method according to ref. 49 . A total of 17.9 ml of KBH 4 aqueous solution (2.0 M, with 0.2 M KOH) was added at a flow rate of 2 ml min −1 to 44.8 ml of 0.2 M Co(CH 3 COO) 2 aqueous solution at 273 K under gentle stirring. When no hydrogen bubbles were released, the black precipitate was stirred at 273 K for additional 30 min for complete reduction. The amorphous Co–B NPs were separated by centrifugation and washed thrice with distilled water, twice with ethanol, twice with PEG200 and finally stored in PEG200 for catalytic testing. The relative molar composition of the amorphous Co–B catalyst is 64.9 Co/35.1 B as determined by ICP–AES. LTFTS In a typical test, the as-leached RQ Fe was dispersed in 20 ml PEG200 and charged into a mechanically stirred 50-ml stainless steel autoclave (CJF-0.05). Then, the reactor was purged three times with syngas (H 2 /CO/N 2 =64/32/4, volume ratio) from a pressurized aluminum cylinder to replace the air, and then filled with the syngas to a pressure of 30 bar at RT of 288 K. Stirring (800 r.p.m.) was commenced on reaching the desired reaction temperature, and on site carbidation was continued for 20 min. The carbided catalyst was separated from the liquid phase by a magnet, washed with ethanol and PEG200 twice and then subjected to activity evaluation under reaction conditions described above [35] . For cobalt catalysts, the catalytic data were collected directly on the as-prepared catalysts. The time-dependent CO conversion was monitored by terminating the reaction at a series of pressures, followed by analysing the CO concentration in the gas phase gas chromatographically. The initial catalytic activity, r 0 , defined as numbers of moles of converted CO per mole of Fe or Co per hour, was determined from the initial reaction rate by extrapolating the slope of the conversion–time curves of CO to zero reaction time. The details in the calculation of the activity were described in Supplementary Methods . The selectivities to CO 2 and hydrocarbons on the RQ Fe catalyst were determined when the total pressure was decreased to ~30 bar during LTFTS. The autoclave was then cooled down to RT. H 2 , N 2 , CO, CH 4 , and CO 2 in the gas phase were analysed by a GC9560 gas chromatograph with a 2-m-long TDX-01 packed column connected to a thermal conductivity detector (TCD) using N 2 as the internal standard. The hydrocarbons in the gas phase (C 1 –C 4 ) were analysed by a GC9160 gas chromatograph with a PONA capillary column (50 m × 0.25 mm × 0.50 μm) connected to a flame ionization detector (FID). The liquid products were extracted by cyclohexane and analysed by the GC9160 gas chromatograph with the PONA capillary column connected to a FID using decahydronaphthalene as the internal standard. The catalysts were tested at least in duplicate. The hydrocarbon selectivities were calculated on carbon basis with the exception of CO 2 . The carbon balance of the FTS products is better than 95%. Ex situ XRD set-up For phase composition determination, the as-leached RQ Fe and the RQ Fe after LTFTS were always protected by PEG200 to avoid oxidation. The conventional XRD pattern was acquired on a Bruker AXS D8 Advance X-ray diffractometer using Ni-filtered Cu K α radiation ( λ =0.15418, nm). The tube voltage was 40 kV, and the current was 40 mA. The 2 θ angles were scanned from 30° to 90°. The synchrotron radiation XRD pattern was collected on a Huber5021 six-circle diffractometer at BL14B1 beamline of the Shanghai Synchrotron Radiation Facility (SSRF). The X-ray beam wavelength ( λ ) was set to 0.12398, nm by a Si (111) channel-cut monochromator. The diffraction intensities were recorded from 20° to 55° at the rate of 1° min −1 with the step of 0.02°. The synchrotron XRD pattern was then converted to 2 θ values corresponding to Cu K α radiation to facilitate a direct comparison. In situ XRD setup The in situ XRD pattern was acquired on a Bruker AXS D8 Advance X-ray diffractometer using Ni-filtered Cu K α radiation ( λ =0.15418, nm). The tube voltage was 40 kV, and the current was 40 mA. The samples were mounted in the in situ cell and heated at 443 K in flowing syngas (H 2 /CO/N 2 =64/32/4, 20 ml min −1 ) at 5 bar. The 2 θ angles were scanned from 32° to 47° at the rate of 1° min −1 with the step of 0.014°. EXAFS analysis The Fe K-edge XAFS data were acquired in the transmission mode at RT on the 1W1B beamline of the Beijing Synchrotron Radiation Facility (BSRF). The beamline was equipped with a Si (111) double crystal monochromator, and the ionization chambers were used to detect the incident and transmitted beam signals. The typical electron beam energy was 2.5 GeV, and the current was 200 mA. The EXAFS data were analysed by the IFEFFIT data analysis package according to the standard procedures [54] . The background was removed by extrapolating the pre-edge region onto the EXAFS region, and the χ ( E ) data were normalized with respect to the edge jump step using the Athena program of the IFEFFIT package. The normalized χ ( E ) was transformed from energy space to k -space with χ ( k ) multiplied by k 1 to compensate for the contributions from light scatters. Subsequently, the k 1 χ ( k ) data in k -space ranging from 3.1 to 13.5 Å −1 were Fourier-transformed to the R -space. The processed χ ( k ) data were fitted in R space ranging from 1.3 to 3.7 Å using the Artemis program of the IFEFFIT package [54] . From these analyses, structural parameters including coordination number ( N ), coordination distance ( R ), Debye-Waller factors and inner potential correction (Δ E 0 ) were obtained. Theoretical RDFs of the ε -Fe 2 C, ε ′-Fe 2.2 C, χ -Fe 5 C 2 and θ -Fe 3 C phases were calculated using the FEFF8.2 code [55] and the crystal structure parameters of these iron carbides compiled in Supplementary Table 1 as the input data. 57 Fe Mössbauer spectroscopy 57 Fe Mössbauer spectroscopy is a powerful tool in identifying and quantifying the iron phases formed in FTS [56] . It is advantageous to XRD in getting access to very small or amorphous iron phases [5] , and advantageous to EXAFS in affording structure-specific information for coexisting iron phases. The 57 Fe Mössbauer spectrum was collected on a spectrometer constructed by the Key Laboratory of Nuclear Analysis Techniques, Chinese Academy of Sciences, using a 57 Co/Rh irradiation source in the constant acceleration transmission mode at RT. The velocity was calibrated by a 25 μm-thick α -Fe foil, and the IS value was referenced to α -Fe at RT. The spectrum was fitted using a least-squares fitting routine that models the spectrum as appropriate superpositions of quadruple doublets and magnetic sextets with Lorentzian line-shape and constrains in peak width and intensity using the MossWinn 3.0i program. The line drawn through the data points is the result of the computer fit. The phase compositions were determined by the areas of the absorption peaks with the assumption of the same recoil-free factor (the probability of absorption of the γ photons) for all kinds of iron nuclei in the catalyst. How to cite this article: Xu, K. et al . ε -Iron carbide as a low-temperature Fischer–Tropsch synthesis catalyst. Nat. Commun. 5:5783 doi: 10.1038/ncomms6783 (2014).